Similarity of wet granular packing to gels To date, there is still no general consensus on the fundamental principle that governs glass transition. Colloidal suspensions are ordinarily utilized as model systems to study the dynamical arrest mechanisms in glass or gels. Here, we tackle the problem using athermal granular particles. Slow dynamics and structural evolution of granular packing upon tapping are monitored by fast X-ray tomography. When the packing are wet and short-range attractive interactions exist, we find a large amount of locally favoured structures with fivefold symmetry, which bear great structural similarity to colloidal gels. In addition, these structures are almost absent in dry packing with similar packing fractions. The study leads strong support for the geometrical frustration mechanism for dynamic arrest in both thermal and athermal systems with attractive interactions. It also suggests nontrivial structural mechanism, if exists, for dynamic arrest in systems with purely repulsive interactions. Random granular packing have been used as archetypical models for disordered hard sphere packing to simulate the structures of liquids and glasses since Bernal [1] . Later, the compaction dynamics of granular packing under mechanical agitations has also been studied similarly to the slow glassy relaxation in thermal glassy systems [2] , [3] . Many insights have been gained in the study of the structure and dynamics based on the glass or jamming paradigm [4] , [5] , [6] . However, almost all existing studies of granular packing drawing analogy with glass physics have been devoted to dry ones. A small amount of liquid inside a granular packing can drastically change its mechanical strength, which is crucial for many practical applications and soil mechanics studies [7] , [8] . Previous studies on dense wet granular packing have focused on the mechanical properties, gas–fluid transition [9] and capillarity effects [10] , [11] , [12] with few experimental studies over the underlying structure [13] , [14] or its possible relationship with glass transition. However, when the capillary attractive force is much larger than the particle weight, it is reasonable to assume that the attractive force can have a great impact on the underlying structure and dynamics. Indeed, the very porous and heterogeneous wet packing bear great similarity with a colloidal gel. As a result, the structure and compaction dynamics of wet granular packing should resemble those of attractive glassy systems as the competition result of bonding and caging effects [15] . Until now, this resemblance has been barely noticed. In this paper, we study the structural evolution of wet granular packing upon tapping using high spatial-resolution synchrotron X-ray microtomography. We analyse the structures using free volume, contact number, pair correlation and high-order angular distribution functions. We find clear differences in the local structures between wet and dry packing. To explain these differences, we find the wet packing consist of a large amount of locally favoured structures (LFSs) with fivefold symmetry, which are almost absent in dry ones. These results suggest the possible different dynamical arrest mechanism for systems with and without attractive interactions. In addition, it also suggests that small local structural changes only involving high-order structural correlations could be responsible for dynamical arrest in glassy systems. Free volume and contact number In dry granular materials, the compaction process has been understood in the statistical framework of Edwards’ ensemble theory, which draws many parallels to thermal glassy systems [2] , [3] . In Edwards’ framework, the volume plays the role of energy [6] . The slow compaction dynamics can be explained using models based on free volume theory or empirical stretched-exponential behaviour [2] . Following previous studies [2] , [3] , [16] , we first obtain the volume fraction φ by analysing the reconstructed packing structures ( Fig. 1 ), then we monitor its change as a function of tapping number as shown in Fig. 2 . The corresponding φ evolves from 0.39 to 0.58 and 0.55 for 12 and 8 g, respectively after 5,000 taps. Unlike in dry packing [2] , [3] , φ shows dramatic increase during the initial several taps. This is consistent with the observation that the initial packing structure has a lot of pores inside, which can easily collapse upon tapping. As the collapse involves the breakage of limited number of capillary bonds, it suggests that volume cannot play exactly the same role as in dry packing. To verify the difference with a dry packing structure, we analyse the probability distribution function (PDF) of the free volume V obtained by standard Voronoi tessellation, as shown in Fig. 3a . In previous study of dry packing [17] , the PDFs of V with φ ranging from 0.55 to 0.64 can be nicely collapsed onto a universal k-Gamma distribution with k ranging from 12.2 to 14.5 (ref. 17 ). As shown in Fig. 3b , similar to dry packing, we rescale the PDFs of V and found they are not well fitted by k-Gamma function for low- φ packing because of the long tails induced by the large pore structures [18] ; when φ is above 0.55, the distribution approaches k-Gamma distributions with k about 10.9±0.5, and the distribution can almost collapse with the dry ones. 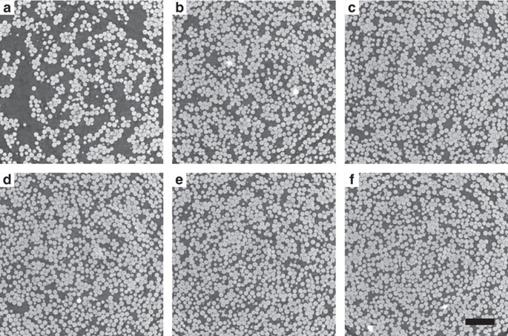Figure 1: Cross-sections of the wet granular packing. (a–f) The cross-sections after 0, 10, 40, 100, 1,000 and 5,000 taps, respectively. The corresponding volume fractionsφin each packing are 0.386, 0.528, 0.553, 0.559, 0.577 and 0.579, respectively. Length of scale bar in panel (f) is 1 mm. Figure 1: Cross-sections of the wet granular packing. ( a – f ) The cross-sections after 0, 10, 40, 100, 1,000 and 5,000 taps, respectively. The corresponding volume fractions φ in each packing are 0.386, 0.528, 0.553, 0.559, 0.577 and 0.579, respectively. Length of scale bar in panel ( f ) is 1 mm. 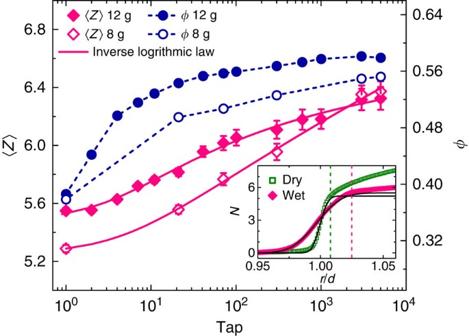Figure 2: Compaction curves. The main panel shows the compaction curves for both volume fractionφand average contact number ‹Z› for wet granular packing with tapping intensity of 12 and 8 g, respectively. The solid lines correspond to the inverse logarithmic fitting according to equation (2). The inset shows the complementary error function fitting to get the average contact number ‹Z› forφ=0.617 dry packing andφ=0.386 wet packing. The error bars forφare smaller than the symbols and the error bars of ‹Z› are determined as two standard deviations from the nonlinear fittings by the complementary error functions. The dashed lines yield contact thresholds 1.008 and 1.025 for dry and wet packing, respectively. Full size image Figure 2: Compaction curves. The main panel shows the compaction curves for both volume fraction φ and average contact number ‹ Z › for wet granular packing with tapping intensity of 12 and 8 g, respectively. The solid lines correspond to the inverse logarithmic fitting according to equation (2). The inset shows the complementary error function fitting to get the average contact number ‹ Z › for φ =0.617 dry packing and φ =0.386 wet packing. The error bars for φ are smaller than the symbols and the error bars of ‹ Z › are determined as two standard deviations from the nonlinear fittings by the complementary error functions. The dashed lines yield contact thresholds 1.008 and 1.025 for dry and wet packing, respectively. 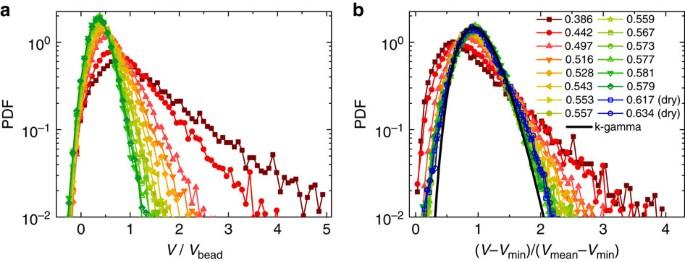Figure 3: Distribution of free volumeV. (a) Probability distribution function of free volumeVfor different tapping numbers. (b) Normalized probability distribution function ofVand k-Gamma fitting for different tapping numbers of wet packing and two dry ones.Vminis the minimum attainable volume andVmeanis the average volume at each tap number. Full size image Figure 3: Distribution of free volume V . ( a ) Probability distribution function of free volume V for different tapping numbers. ( b ) Normalized probability distribution function of V and k-Gamma fitting for different tapping numbers of wet packing and two dry ones. V min is the minimum attainable volume and V mean is the average volume at each tap number. Full size image We also analyse the evolution of the average contact number ‹ Z ›. In low-density wet granular packing, the particles are held together by capillary bonds instead of being confined by the cages formed by their neighbours. Thus, it is more reasonable to study the local structures based on ‹ Z › using the bonding picture, similar to that in colloidal gel case [15] . However, as φ increases, we would expect caging effect will play an increasingly important role. In obtaining the average contact number ‹ Z ›, we adopt a similar technique as in the analysis of the contact number in dry granular packing by fitting the evolution of neighbour number N as a function of a normalized minimum distance parameter using a complementary error function [19] where d is the particle mean diameter, ξ is the contact variance and ‹ Z › is the average contact number that needs to be fitted. As shown in the inset of Fig. 2 , the function for a wet packing shows a large spread at contact as compared with that of a dry one owing to the existence of finite-length capillary bonds, which can generate a spread in the inter-particle distances. We adopt a contact threshold of 1.025 d so that the average contact number is consistent with the fitted value. The threshold value is reasonable after taking into account the average liquid bond volume and the critical breakage length [20] . The corresponding contact threshold is found to be 1.008 d for dry granular packing. The compaction curves of ‹ Z › are shown in Fig. 2 which look quite different from those of φ . Instead, they are similar to the compaction curve of φ in dry packing [3] . We find the compaction curves of ‹ Z› fit well with an inverse logarithmic law [3] (shown in Fig. 2 ), where is the initial average contact number, is the final average contact number, τ is a characteristic time, t is the tapping number and B is a fitting parameter. The good fitting indicates a bonding-controlled activation dynamics is in effect [16] . Correlation functions To understand the clearly different compaction dynamics of a wet packing, we analyse several correlation functions of the local structures of both wet and dry packing. We first analyse the pair correlation function g(r) as shown in Fig. 4a . The significant differences emerge in the initial several taps, of which g(r) decreases significantly in the r range of (1.6 d –1.75 d ), which are noted later as corresponding to the decrease of the number of bipyramids ( r =1.63 d ). The g(r) of dry packing is clearly lower in the same range even at high density. It suggests that some local structural motifs are more populous in wet packing. When r >2.5 d , correlation disappears for both dry and wet packing implying that both of them are structurally short-ranged correlated and most of the structural differences are within the first coordination shell. 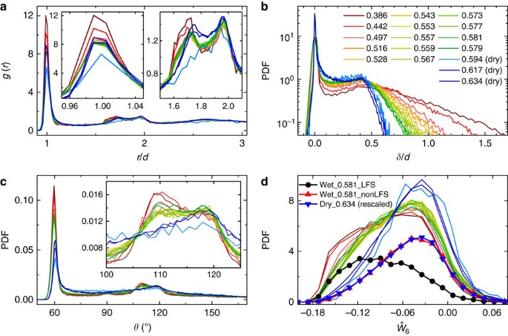Figure 4: Correlation functions. (a) Pair correlation functiong(r). Insets show the magnified distributions around the peaks ofg(r). (b) Surface-to-surface distance distribution function. (c) Angular distribution function. The inset shows the magnified second peak. (d)bond order parameter distribution. Lines with filled circle and up-triangle symbols correspond to contributions from LFS-like structures and not, respectively, inφ=0.581 wet packing. Line with filled down-triangle symbols is thedistribution forφ=0.634 dry packing after rescaled to have the same magnitude as that of non-LFS-like structures inφ=0.581 wet packing. They almost collapse with each other. Figure 4: Correlation functions. ( a ) Pair correlation function g ( r ). Insets show the magnified distributions around the peaks of g(r) . ( b ) Surface-to-surface distance distribution function. ( c ) Angular distribution function. The inset shows the magnified second peak. ( d ) bond order parameter distribution. Lines with filled circle and up-triangle symbols correspond to contributions from LFS-like structures and not, respectively, in φ =0.581 wet packing. Line with filled down-triangle symbols is the distribution for φ =0.634 dry packing after rescaled to have the same magnitude as that of non-LFS-like structures in φ =0.581 wet packing. They almost collapse with each other. Full size image In wet packing, the contact peaks of g(r) around r = d are wider and decline more steeply on the right side as compared with dry packing. To visualize this more clearly, we also plot the particle surface-to-surface distance δ distributions in Fig. 4b . The wider contact peaks in wet packing correspond to particles held together by capillary bonds and the much steeper decline of the contact peak is clearly due to particles being shielded by contacting neighbours. This is consistent with the fact that the wet packing tend to have a larger ‹ Z › about 6.3 at φ =0.581 (refs 14 , 21 ), to be compared with 5.5 at φ =0.617 and 5.8 at φ =0.634 in dry packing. This behaviour has been observed in a recent study on attractive emulsions despite a large polydispersity effect [22] . As g(r) only provides two-body correlation information, we go beyond it by analysing higher-order correlation functions. In Fig. 4c , we analyse the angular distribution function that corresponds to the distribution of angular distances between two particles, which are in contact with the same particle. The differences between dry and wet packing are more pronounced in angular distributions. The major differences are located at 60° and 109°. The 60° peak corresponds to equilateral triangle of particles, which suggests that two particles in contact with a central particle are more likely to be in contact with each other in wet packing. The peak around 109° corresponds to the appearance of bipyramids. The 120° peak corresponds to a diamond structure, which is shared by both dry and wet packing. There is a very subtle evolution of the peak height at 109°: it is high at the low-density packing and decreases first and then rises again. This can be explained by the nontrivial evolution of the number of bipyramids inside the packing as shown later. Locally favored structures The clearly different local structures between dry and wet packing indicate the existence of some different local structural motifs and possible different mechanisms for dynamical arrest. The mechanism of glass transition has been under extensive investigations for decades [23] . Not without controversy, proponents aiming at structure mechanisms have suggested polyhedral order [24] , [25] , [26] , crystalline order [27] , [28] or point-to-set type of amorphous order [29] , [30] as the possible candidates for dynamical arrest. The polyhedral order normally cannot tile the Euclidean space. Similar to previous searches for aforementioned orders in dry packing [31] , we have calculated the Q 4 , Q 6 and bond order parameters to identify the possible crystal-like orders and fivefold symmetries for both dry and wet packing [24] (see Methods). It turns out that there exists no local crystal order for both dry and wet packing from Q 4 and Q 6 distributions. This is in contrast with a recent study on colloidal hard spheres [32] and in agreement with a previous study on dry granular packing [19] . In Fig. 4d , we show the distribution. Unlike Q 4 and Q 6 distributions (not shown), the distributions of wet packing have large shifts towards negative values compared with those of dry ones, which suggests the possible existence of fivefold symmetry structures [32] . In the following, we identify the existence of some local polyhedral structural motifs as LFSs directly to explain the different local structures found in wet packing [33] , [34] . The structures only account for particles in contacts including contacts by liquid bonds. Following the notation in ref. 34 , the major LFSs we obtain include 5A (bipyramid), 6A (octahedron), 6Z, 7A (pentagonal bipyramid) and so on, as shown in Fig. 5a . Larger LFSs with more particles in the clusters are almost absent. If a bead is shared by two types of LFSs, we identify it to belong to the larger one (see Methods). 5A, 6Z and 7A are consistent with the fivefold symmetry and 6A is part of face-centred cubic (fcc) structure. However, the number of 6A remains rather small and constant over the whole compaction process. This is contrary to a hard-sphere colloidal study in which crystal-like order is more populous than local order with fivefold symmetries [32] . We calculate the total fraction of beads involved in these LFSs for different tap numbers and show it in Fig. 5a,b for tapping intensity 12 and 8 g, respectively. The fraction shows nontrivial evolution during compaction. It has a value around 52% in the initially prepared packing, then it decreases to around 38% and rises again at φ ≈0.55. This is close to that of random loose packing φ RLP when the particles start to feel strongly the caging effects from its neighbours. The final compactified packing with φ ≈0.58 is therefore a state when both caging and bonding effects are important. For comparison, we also calculate the LFSs in dry packing and find they are almost nonexistent (2.8%) if we limit the structures to contacting neighbours only. Even if we artificially increase the threshold distance to 1.025 d for dry packing to include more particles as contacting neighbours, we can still only find less than 13% of particles in the LFSs, which is compared with the 50% in wet ones (these two fractions are indicated by two dashed lines in Fig. 5a in comparison to wet packing). The existence of large quantities of the LFSs suggests that system with attractive forces will form some real-space structural motifs upon dynamical arrest, which might be relevant to dynamical slowing down [34] . We also find that particles in LFSs have more bonding neighbours as compared with particles not in LFSs, as shown in Fig. 5c , which indicates that these structures are energetically preferred as more bonds correspond to lower energy. 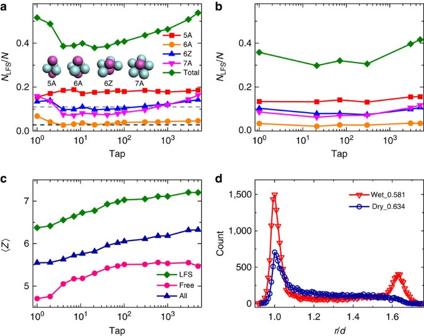Figure 5: Locally favoured structures. (a) The fraction of LFSs inside the wet packing as a function of tapping number at tapping intensity of 12 g. The dark and light dashed lines correspond to fraction of LFSs insideφ=0.617 dry packing when the threshold distances are chosen as 1.008dand 1.025d, respectively. (b) The fraction of LFSs inside the wet packing as a function of tapping number at tapping intensity of 8 g. (c) Average contact number ‹Z› of particles inside LFSs and not. (d) Distribution of the distances of spindle particles in CCN3s as defined in Methods section. Figure 5: Locally favoured structures. ( a ) The fraction of LFSs inside the wet packing as a function of tapping number at tapping intensity of 12 g. The dark and light dashed lines correspond to fraction of LFSs inside φ =0.617 dry packing when the threshold distances are chosen as 1.008 d and 1.025 d , respectively. ( b ) The fraction of LFSs inside the wet packing as a function of tapping number at tapping intensity of 8 g. ( c ) Average contact number ‹ Z › of particles inside LFSs and not. ( d ) Distribution of the distances of spindle particles in CCN3s as defined in Methods section. Full size image To interpret the above results, we draw analogies with colloidal physics despite the athermal nature of granular packing. In colloidal community, the low- φ phase formed by systems with short-range attractive interaction is called a gel, which results from arrested phase separation [35] , [36] . The high- φ phase could be a dense gel/attractive glass or a repulsive glass depending on the ratio between interaction energy and temperature [37] , [38] . In our case, as capillary attractive force of the liquid bridge is several hundred times of the gravity of a bead, the fate of the high- φ phase, therefore, is most likely a dense gel/attractive glass. The extensive stirring in the preparation of the low- φ packing in the beginning is similar to quenching the system from a high temperature to form a gel with ‘liquid–gas’ coexistence. The large pores correspond to the ‘gas’ phase and the dense particle network is similar to the ‘liquid’ percolating network of a gel. As shown before, the compaction at a constant tapping intensity facilitates the phase separation by removing the ‘gas’ phase until the system reaches rather high φ . This corresponds to a pure ‘liquid’ in gel, which is arrested into either attractive glass or repulsive glass [35] . As noted before, it is most likely an attractive one. To support the above scenario, we resort further to a structure argument to demonstrate the intrinsic analogy of these two systems. It turns out the microscopic structure of our wet packing is quite similar to that of a colloidal gel by Royall et al. [34] Especially, if we compare our φ =0.385 packing with φ =0.35 colloidal gel [34] , we find that not only the average contact number ‹ Z ›, but also the fraction and types of LFSs are similar. This strongly suggests the analogy between a wet granular packing and a gel is not superficial and is deeply related owing to a possible shared dynamic arrest mechanism of structural origin. However, we do notice there exists some differences: first, there exists far less population of 6A in wet granular packing as compared with the colloidal gel [34] which corresponds to fcc structure. Recently, bond orientational orders based on crystalline symmetry have gained quite popularity as the potential dynamic arrest mechanism for glass transition [27] . Our current work, on the other hand, suggests a different dynamic arrest mechanism might be at work as our system is abundant in LFSs with fivefold symmetry instead of crystalline ones [32] , [34] . Second, in our wet packing, the distributions have substantial shifts towards negative values as compared with the dry ones. We can separate the distributions into contributions from LFS-like structures and not (see Fig. 4d ). The separation is clear and strongly supports the existence of corresponding LFSs. In the corresponding colloidal work [34] , the distribution does not contain such distinctive features, and the identifications of LFSs are based on theoretical presumptions. Based on the above interpretations, several important conclusions can be drawn. First, the resemblance of the local structures of the arrested high- φ packing with those of their low- φ counterparts corroborates the phase-separation scenario for gelation. Second, the rather different structures of the high- φ wet packing from the dry ones of similar φ suggest that they should be considered more like attractive glasses instead of repulsive ones. Currently, there exists great interest from the gel community to understand the nature of the phase-separated dense phase when both caging and bonding effects are important [35] , [36] . In our study, extensive tapping in reaching the high- φ packing corresponds to a rather long structural relaxation time. The different local structures of packing with and without attractive interactions at similar φ suggest that the bonding effect is still dominating over the caging effect in determining the local structures [36] . This also demonstrates in an indirect way the importance of attractive forces for glass transitions [37] , [39] . Last and most important, the abundance of fivefold symmetry real-space structures in wet granular packing brings strong support for the geometric frustration mechanism for dynamical arrest [25] , [26] , [40] . And the apparent lack of corresponding LFSs in dry packing suggests that if such real-space structures exist in dry ones, they will inevitably be of a different kind [31] . Overall, one thing worth emphasis is that all the aforementioned differences are hardly discernable in simple pair correlation functions and free volume distributions. It therefore highlights the importance of studying high-order structural correlations and small local structural changes to understand their connections to dynamical arrest in glassy systems [41] . As noted above, to detect high-order structural correlations and subtle structural transformations, direct real-space study will be more relevant than statistically averaged methods. Until now, colloids have been the ideal ‘atoms’ to test all hypotheses related to dynamically arrested phases like gels [34] , [35] , [42] , [43] , [44] . In the current study, we suggest that wet granular materials can serve as suitable complements for similar investigations. Despite the fact that granular particles are by nature athermal and with frictions, the study of them has several advantages: first, it is convenient to choose the right-size granular particles to match the experimental imaging resolution, which can enhance the detection efficiency of very subtle structural features as noted above. This is crucial when these features can easily be overwhelmed by thermal noises. Second, granular packing can be prepared with large packing fractions close to the random close packing, which are hardly accessible for both simulations and colloidal experiments. This can be useful for their applications in deep quenched glassy phases. We do note that coherent synchrotron scattering techniques especially those based on free electron laser might offer the final solution for the structural problems in atomic and molecular systems. Experiments Glass beads ( d =200±15 μm, Duke Scientific) are mixed with aqueous solution of potassium iodine (17 μl) to form a mixture in which the volume ratio between the liquid and particles is 0.033. At this volume ratio, the liquid forms mostly as binary capillary bonds between the particles. It is estimated that the liquid bridge capillary force is several hundred times of the gravity of a bead. The mixture is stirred extensively using a plastic rod in a clean Petri dish to make the liquid uniformly distributed. Then, it is gently poured into an acrylic cylindrical container (ID=9.6 mm) to a height about 15 mm. The packing is compactified using an electromagnetic exciter, which can generate pulse taps. Each tap consists of a single cycle of 30-Hz sine wave at 12 g peak-to-peak acceleration. We also carry out a similar study at 8 g tapping intensity. The results are in general agreement with those of 12 g. Successive taps are spaced with 1/3 s intervals to allow the system to relax. The structural evolutions of the packing are studied by a synchrotron fast X-ray microtomography setup at 2-BM beamline of the advanced photon source of Argonne National Lab. A complete tomographic scan includes 1,800 projection images recorded in a course of 6 s. The size of the projection image is 2,016 (H) × 1,200 (V) pixels with an effective pixel size of 5.5 μm. About 3.5 mm length at the middle of the wet packing is recorded at many different tap numbers with a maximum of 5,000 taps (the cross sections are shown in Fig. 1 ). The dry packing are prepared using the same beads by tapping at different intensities for 1,000 times in reaching different volume fractions φ =0.617 and 0.634. The φ =0.594 packing is drawn from another study with the packing generated by ‘raining’ the particles from a sieve, which has only about 2,000 particles inside, therefore with less statistics compared with other packing. Owing to different absorption rates of X-rays, the air, glass beads and liquid show different grey-scale values in the reconstructed three-dimensional images, which can be used to segment the images in obtaining each particle’s size and position with error less than 0.02 d . About 10,000 particles within an inner diameter of 7.2 mm of the container are analysed to avoid the boundary effect. Bond orientational order To identify the ordering structures such as icosahedron, fcc and hexagonal close-packed, we calculate several bond orientational order parameters defined as following: where the coefficients are Wigner 3J symbols and where Y lm are spherical harmonics [24] and the average is taken over particles of which distances from central particles are less than 1.4 d . To evaluate the possible influence of number of neighbours over the bond orientational order parameters [45] , we also use a cutoff distance of 1.2 d to calculate all bond orientational order parameters. No qualitative changes in the distributions have been found other than a slight shift in the values. We therefore believe the calculation results are robust. Procedure to find LFSs The LFSs in our system turn out to be 5A, 6Z, 7A and 6A. We first find all pairs of particles (spindle particles) that have three (CCN3), four (CCN4) or five (CCN5) common contacting neighbours. A perfect bipyramid (5A) corresponds to a CCN3 where the distance between spindle particles equals exactly 1.63 d . We therefore calculate the distributions of the distances of spindle particles for all CCN3s in our wet and dry packing as shown in Fig. 5d . We find that there exists a significant peak at 1.63 d for wet packing and not for dry packing. This suggests that 5A is one of the LFSs in the wet packing. This peak in Fig. 5d is also consistent with the peak at 109° in angular distribution function from simple geometric calculations of bipyramids ( Fig. 4c ). Taking into account the polydispersity and the uncertainties of particle centres brought by image processing, we select the CCN3s whose distances between spindle particles are in the range of (1.61 d –1.65 d ) as 5A, which corresponds to the peak in Fig. 5d . If two 5As share four particles, we denote them as a 6Z. Similar to 5As, we identify octahedrons (6A) from CCN4s by choosing those with spindle particle distances in the range of (1.39 d –1.43 d ). Finally, all CCN5s are identified as pentagonal bipyramids (7A). How to cite this article : Li, J. et al. Similarity of wet granular packing to gels. Nat. Commun. 5:5014 doi: 10.1038/ncomms6014 (2014).